Electrical control of large magnetization reversal in a helimagnet Reversal of magnetization M by an electrical field E has been a long-sought phenomenon in materials science because of its potential for applications such as memory devices. However, the phenomenon has rarely been achieved and remains a considerable challenge. Here we report the large M reversal by E in a multiferroic Ba 0.5 Sr 1.5 Zn 2 (Fe 0.92 Al 0.08 ) 12 O 22 crystal without any external magnetic field. Upon sweeping E through the range of ±2 MV m −1 , M varied quasi-linearly in the range of ±2 μ B per f.u., resulting in the M reversal. Strong electrical modulation of M at zero magnetic field were observable up to ~\n150 K. Nuclear magnetic resonance measurements provided microscopic evidence that the electric field and the magnetic field play equivalent roles in modulating the volume of magnetic domains. Our results suggest that the soft ferrimagnetism and the associated transverse conical state are key ingredients to achieve the large magnetization reversal at fairly high temperatures. Electric-field ( E ) control of magnetization ( M ) has certain advantages over current-driven control because of its smaller power consumption. For several decades, the capability of achieving this type of control has been tested in a special class of magnetic insulators, so-called magnetoelectrics (MEs) or multiferroics, in which M (or the electric polarization P ) is expected to be modulated by E (or the magnetic field H ) [1] , [2] , [3] . Such cross-coupling effects between the magnetic and electric order parameters can be effectively described in terms of direct and converse magnetoelectric effects [4] : where α ( α c ) and β ( γ ) represent the linear and quadratic ME (converse ME) coefficients. If any of the above direct ME coefficients is large, significant converse ME effects should be observable, as the two types of effects are roughly proportional to each other. However, most ME and multiferroic compounds have thus far exhibited quite small ME coefficients such that the modulation of M by E is too small to be practically useful [5] , [6] , [7] . It is only recently that several multiferroic compounds have demonstrated appreciable modulation of M with enhanced ME coupling coefficients [8] , [9] , [10] . On the other hand, to better exploit ME multiferroics in practical devices, for example, magnetic information storage, M reversal by E without the application of an H -bias becomes a key requirement. Very recently, there has been progress towards achieving this goal. The reversal of ferromagnetic domains has been successfully achieved in a ferromagnet/multiferroic heterostructure at room temperature [11] . However, the observation was limited to interface magnetism. Tokunaga et al. [12] have demonstrated bulk magnetization reversal in Dy 0.75 Gd 0.25 FeO 3 and Dy 0.7 Tb 0.3 FeO 3 at 2.5 K, with a maximum modulation of ~\n±0.2 μ B per f.u. However, full reversal could be achieved only at very low temperatures—below 3 K—because the phenomenon stems from the coupling between rare-earth and Fe moments. Meanwhile, magnetization reversal has been demonstrated in an archetypal ME Cr 2 O 3 crystal at room temperature, but the modulation strength was small (10 −3 emu g −1 , equivalent to ~\n3 × 10 −5 μ B per f.u.) [13] because of the small ME coefficient, as is typically observed in linear MEs [5] . Therefore, it is highly desirable to search for a novel mechanism that can drive bulk magnetization reversal with large modulation amplitudes, high switching speeds and high operation temperatures. To this end, we note that ferrites with hexagonal structures have several advantages. Such systems have long been used in applications such as refrigerator magnets and floppy disks because of their large ferrimagnetic moments and high ordering temperatures [14] . Because of their structural flexibility of the c -axis stacking sequence and chemical substitution, numerous hexaferrites with wide structural variants (M, Y, W, Z, X and U-types) have been identified, and more may potentially be found. More interestingly, when structure and spin frustration are properly controlled, it has been rather recently found that many of these hexaferrites can become ME with stabilization of a helical or conical spin ordering [15] . The first discovery of such ME effects was made by Kimura et al. [16] in a Zn 2 Y-type hexaferrite Ba 0.5 Sr 1.5 Zn 2 Fe 12 O 22 , in which field-induced P was observed at the magnetic field around 1 T. It was subsequently found that the critical magnetic field necessary to induce P became substantially lowered (~\n1–10 mT) in Mg 2 Y-type [17] or Al-doped Zn 2 Y-type hexaferrites, resulting in giant ME coupling [18] . Furthermore, direct ME effects were also observed at fairly high temperatures in M-type hexaferrites [19] and even at room temperature in Co 2 Z-type hexaferrites [20] . Later on, direct ME effects were also found in the new U- and W-type hexaferrites [21] , [22] . Therefore, upon further control of the material properties of these electrically active hexaferrites, it is expected that large converse ME effects may potentially be achieved. In the case of the converse ME effect, strong M modulation by E and four non-volatile M states were first observed at room temperature in a single crystal of Co 2 Z-type hexaferrite, in which the maximum direct ME coupling constants were ~\n3,200 and ~\n150 ps m −1 at finite (=10.5 mT) and zero H -bias, respectively [10] . The modulation of M by E was indeed observed without H -bias at room temperature, but the ME effect was dominantly quadratic, so the reversal of M could not be achieved. Very recently, converse ME effects have also been reported at room temperature in polycrystalline Co 2 Y-type hexaferrites with a maximum converse ME coupling constant of ~\n400 ps m −1 at an H -bias of 1.3 mT [23] . Although nearly linear modulation of M by E was observed, the reversal of M by E could not be achieved without invoking an H -bias. Therefore, to date, the true reversal of M by E without any bias magnetic field has not been achieved in hexaferrites, presumably because of the dominant quadratic modulation and the small ME coupling constants. Moreover, the microscopic mechanism for the realization of large converse ME effects in hexaferrites remains unknown. Here we report the realization of strong modulation and large reversal of magnetization by E in a multiferroic Ba 0.5 Sr 1.5 Zn 2 (Fe 0.92 Al 0.08 ) 12 O 22 crystal at zero H , in which a transverse conical spin state exhibits remanent M and P below ~\n150 K. The strong modulation of M in the range of ±2 μ B per f.u. under the electric-field variation of ±2 MV m −1 was achieved, clearly resulting in the reversal of M up to ~\n100 K. Moreover, the remanent M exhibited non-volatile changes of ±0.11–0.15 μ B per f.u., depending on the history of the applied electric field up to ~\n150 K. NMR measurements showed microscopic evidence that the electric field and the magnetic field play equivalent roles in modulating the volume of magnetic domains. Basic properties of Ba 0.5 Sr 1.5 Zn 2 (Fe 0.92 Al 0.08 ) 12 O 22 Ba 0.5 Sr 1.5 Zn 2 (Fe 0.92 Al 0.08 ) 12 O 22 consists of a series of tetrahedral and octahedral Fe/Zn layers stacked along the c -axis (||[001]) [24] , as shown in Fig. 1a . Under zero-field cooling below 60 K, it is known from neutron-diffraction studies [25] that the compound exhibits an incommensurate longitudinal conical ordering, in which the alternating small ( S ) and large ( L ) magnetic blocks have antiparallel c -axis components and in-plane helical ordering ( Fig. 1b ). On the other hand, under field-cooling process or after the application of μ 0 H ≥0.1 T subsequent to the zero-field cooling, a transverse conical state with a commensurate modulation vector k 0 =(0, 0, 3/2) forms ( Fig. 1c , left). It was also found that the transverse conical state formed at finite H still remains as a metastable phase even after the external H is removed ( Fig. 1c , right). After such an ME annealing procedure (see Methods and Fig. 2a ), the material thus becomes multiferroic, exhibiting remanent M and P -values in the M–H ( Fig. 2b ) and P–H ( Fig. 2c ) hysteresis loops ( P (||[120]) ⊥ M (||[100]) and also in the P–E hysteresis loop ( Fig. 2d ). The ferroelectric phase diagram of this material is summarized in Supplementary Fig. 1 . 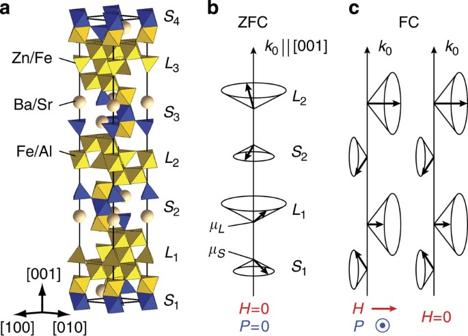Figure 1:Crystal and magnetic structures of Ba0.5Sr1.5Zn2(Fe0.92Al0.08)12O22. Schematic diagrams of (a) the crystal structure, (b) the longitudinal conical spin state formed after zero-field cooling (ZFC), and (c) the transverse conical spin state formed after field cooling (FC).μLandμSdenote the net magnetic moments in theLandSblocks, respectively, andk0is the spin modulation vector. Figure 1: Crystal and magnetic structures of Ba 0.5 Sr 1.5 Zn 2 (Fe 0.92 Al 0.08 ) 12 O 22 . Schematic diagrams of ( a ) the crystal structure, ( b ) the longitudinal conical spin state formed after zero-field cooling (ZFC), and ( c ) the transverse conical spin state formed after field cooling (FC). μ L and μ S denote the net magnetic moments in the L and S blocks, respectively, and k 0 is the spin modulation vector. 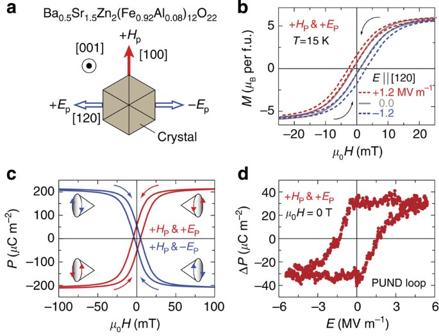Figure 2:Basic properties of Ba0.5Sr1.5Zn2(Fe0.92Al0.08)12O22after the magnetoelectric annealing procedures. (a) A schematic diagram of the ME annealing schemes of +Hp& +Epand +Hp& −Ep.HpandEpdenote the magnetic and the electric poling fields applied during the ME annealing procedures, respectively. (b)M–H, (c)P–Hand (d)ΔP–Eloops of Ba0.5Sr1.5Zn2(Fe0.92Al0.08)12O22at 15 K. The spin helicity of the transverse conical state and the resultant electric-polarization direction are most likely determined by the ME annealing conditions, represented by +Hp& +Epor +Hp& −Ep(see Methods for a description of the procedures). TheΔP–Ehysteresis loop, based on the Positive-Up-Negative-Down (PUND) method, indicates that the sample is ferroelectric atH=0 after being subjected to ME annealing (+Hp& +Ep). Full size image Figure 2: Basic properties of Ba 0.5 Sr 1.5 Zn 2 (Fe 0.92 Al 0.08 ) 12 O 22 after the magnetoelectric annealing procedures. ( a ) A schematic diagram of the ME annealing schemes of + H p & + E p and + H p & − E p . H p and E p denote the magnetic and the electric poling fields applied during the ME annealing procedures, respectively. ( b ) M–H , ( c ) P–H and ( d ) ΔP–E loops of Ba 0.5 Sr 1.5 Zn 2 (Fe 0.92 Al 0.08 ) 12 O 22 at 15 K. The spin helicity of the transverse conical state and the resultant electric-polarization direction are most likely determined by the ME annealing conditions, represented by + H p & + E p or + H p & − E p (see Methods for a description of the procedures). The ΔP–E hysteresis loop, based on the Positive-Up-Negative-Down (PUND) method, indicates that the sample is ferroelectric at H =0 after being subjected to ME annealing (+ H p & + E p ). Full size image In the M–H hysteresis loops, M is easily saturated and changes sign at small H values of ~\n±30 mT with a small coercive field of ~\n2 mT, indicating that Ba 0.5 Sr 1.5 Zn 2 (Fe 0.92 Al 0.08 ) 12 O 22 is a very soft ferrimagnet in the transverse conical state. Very small magnetic anisotropy in the ab -plane is also confirmed by the angular dependence of P under the horizontal rotation of H (see Methods and Supplementary Fig. 2 ). The P–H hysteresis loops also demonstrate the saturation and sign change of P at ~\n±40 mT, which is similar to the scale of the field required for M reversal. The overall shapes of the M–H and P–H loops thus appear similar to each other. The observations suggest that the soft ferrimagnetic domains and the associated ferroelectric domains must coincide each other, as has similarly been claimed to occur in CoCr 2 O 4 (ref. 26 ). In the P–H hysteresis loops, it is also apparent that a saturated P changes sign upon a change in the initial direction of electric poling ( E p ) during the ME annealing procedure ( Fig. 2a ). The origins of such a finite P , which changes in sign with varying H -bias and E p , and the P ⊥ M relation can be qualitatively understood via the spin current model [27] , [28] , in which P ∝ k 0 × ( μ S × μ L ), where μ S and μ L are the net moments of the adjacent S and L spin blocks, respectively. The sign-changing behaviour of P with variations in the E p direction is therefore likely to induce different spin helicities, defined as Σ μ S × μ L , because the E p direction can energetically fix the local spin current direction, μ S × μ L . It is also important to note that the nearly linear variation of P at a small H -bias facilitates the production of the highest ME coefficient (d P /d H ) of ~\n15,000 ps m −1 at zero H among bulk multiferroic compounds [18] . Therefore, it is expected that a large converse ME effect should be observed in this compound, although no experimental investigation has yet been conducted. 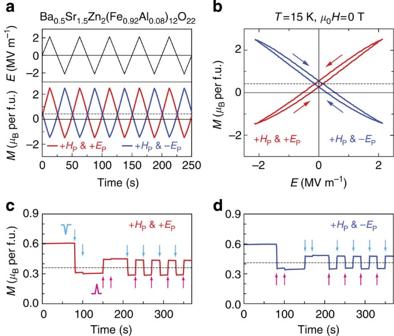Figure 3: Repeatable, strong modulation and large reversal of magnetization by electric fields. (a) Periodic modulations ofM||[100] at zero magnetic field under repeating triangular waves ofE||[120] after the ME annealing. (b) The resultantM–Eloops illustrating the reversal; the magnetization was initially at ~\n0.6 μBper f.u. because of the +Hpcondition, and its average value was ~\n0.4 μBper f.u. (dotted lines). (c,d) Jumps in the remanentMcaused by a short, triangular electric pulse with either a positive (red arrows) or negative (blue arrows) peak value of 6.8 MV m−1and a duration of 0.5 ms for the two ME annealing conditions of (c) +Hp& +Epand (d) +Hp& −Ep. The magnetization, which was measured for ~\n0.1 s per point, appears to have changed immediately upon application of the short electric pulse, and the recorded information regarding the pulse history is non-volatile. Electrical modulation and reversal of M at low temperature Figure 3a demonstrates that a giant M modulation can be induced by the application of E at zero H- bias in a Ba 0.5 Sr 1.5 Zn 2 (Fe 0.92 Al 0.08 ) 12 O 22 single crystal. Before any experiment was performed, the transverse conical phase was first stabilized at zero H- bias after ME annealing with the + H p & + E p condition. Then, a slowly varying E ||[120] in the range of ±2 MV m −1 was repeatedly applied with a period of 40 s, while the magnetization M ||[100] was recorded using a vibrating sample magnetometer to measure the magnetization at time intervals of 0.1 s. We observed a gigantic change in M that was approximately proportional to the change in E , with a modulation of Δ M ~\n±2 μ B per f.u. for the sweep of E through the range of ±2 MV m −1 ( Fig. 3a ). It is noteworthy that this modulation of Δ M ~\n±2 μ B per f.u. represents the largest modulation magnitude ever observed in a bulk compound. The average value of M at zero H -bias in this repeated measurement was ~\n0.4 μ B per f.u., indicating that M varied between 2.4 and −1.6 μ B per f.u., demonstrating the unambiguous reversal of the bulk magnetization direction. The quasi-linear modulation of M was repeatable for many cycles of the E sweep, so the resultant M–E loop was quite reproducible ( Fig. 3b ). Interestingly, the M–E loops exhibited a small hysteresis, resulting in two stable remanent magnetization M r values (0.47 and 0.33 μ B per f.u.) at zero E- bias. Upon changing the ME annealing condition to + H p & − E p , the M exhibited a quasi-linear decrease with increasing E (blue lines in Fig 3a,b ), but the full hysteresis loop retained the same two M r values. In other words, M clearly exhibited two non-volatile M r states at zero E- bias, the values of which depended on the history of the E sweep and also the sign of E p in the ME annealing procedure. Figure 3: Repeatable, strong modulation and large reversal of magnetization by electric fields. ( a ) Periodic modulations of M ||[100] at zero magnetic field under repeating triangular waves of E ||[120] after the ME annealing. ( b ) The resultant M–E loops illustrating the reversal; the magnetization was initially at ~\n0.6 μ B per f.u. because of the + H p condition, and its average value was ~\n0.4 μ B per f.u. (dotted lines). ( c , d ) Jumps in the remanent M caused by a short, triangular electric pulse with either a positive (red arrows) or negative (blue arrows) peak value of 6.8 MV m −1 and a duration of 0.5 ms for the two ME annealing conditions of ( c ) + H p & + E p and ( d ) + H p & − E p . The magnetization, which was measured for ~\n0.1 s per point, appears to have changed immediately upon application of the short electric pulse, and the recorded information regarding the pulse history is non-volatile. Full size image Switching of remanent magnetization by electric pulses Figure 3c further demonstrates that the two M r values could be controlled by the application of short E pulses. Figure 3c presents the trace of the M r values, which was initially 0.6 μ B per f.u. after ME annealing under the + H p & + E p condition. Upon the application of a short negative pulse of a triangular E wave with a peak value of 6.8 MV m −1 and a duration of 0.5 ms, the M r value suddenly dropped to 0.3 μ B per f.u. The drop in M r caused by the first E pulse was relatively larger. The second negative pulse induced only a negligible drop in M r , whereas the subsequent positive pulse caused M r to sharply increase once again to 0.45 μ B per f.u. Thus, the sequential application of E pulses of opposite direction resulted in sharp jumps of M r between two independent values centred near 0.37 μ B per f.u., whereas the latter of two successive E pulses of the same sign did not produce any appreciable change in M r . The switching of M r between the two values was well-reproducible after many E pulses, with no evidence of any fatigue effect. Figure 3d presents the trace of the M r values when the ME annealing was performed under the + H p & − E p condition. In this case, the effects of the short positive and negative pulses were reversed, but the overall behaviour was quite similar to that in the case of + H p & + E p condition. The M r values switched between 0.35 μ B per f.u. and 0.47 μ B per f.u., centred on a value of 0.41 μ B per f.u. The ability to induce such non-volatile M r changes through the application of short E pulses implies that the ferroelectric and ferrimagnetic domain configurations at zero H- bias can be tuned by an external electric field, possibly via the microscopic ME coupling inherent to the investigated hexaferrite. It is also noteworthy that the two non-volatile M r values and the ability to switch the remanent magnetism between these two values using short electric pulses could be observed even at higher temperatures. 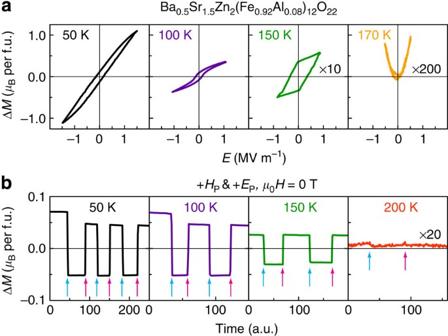Figure 4: High-temperature modulation of magnetization under continuous and pulsed electric fields. (a) ΔM–Eloops measured at 50, 100, 150 and 170 K. Hysteretic modulation was clearly observed up to 150 K (as high as 160 K). The central magnetization values at each temperature were found to be ~\n0.45, 0.48, 0.10, and 0.02 μBper f.u., respectively, and this value was subtracted in each plot to more clearly display the magnetisation behaviour. (b) The non-volatile change in remanentMafter the application of a short, triangular electric pulse with either a positive (red arrows) or negative (blue arrows) peak value of 4.2 MV m−1, demonstrating that theMjumps occurred up to at least 150 K. The zero value at 200 K corresponds to the central magnetization value of 0.03 μBper f.u. Electrical control of magnetization at higher temperatures Figure 4 summarizes the M–E hysteresis loops ( Fig. 4a ) and the variation in M r values caused by short E pulses ( Fig. 4b ) at and above 50 K. The M–E hysteresis loop and the change in M r under short E pulses were clearly observable up to at least 150 K, although the maximum Δ M and the magnitude of the M r jumps systematically decreased with increasing temperature. The temperature window of 150–170 K is consistent with the region in which the phase diagram indicates the stabilization of the transverse conical state only at finite magnetic fields (see Supplementary Fig. 1 ). In particular, at T =170 K, the M–E loop evolved into a combination of linear and quadratic ME behaviours, exhibiting an asymmetric parabolic shape ( Fig. 4a ). Moreover, the hysteretic behaviour became negligible above this temperature, and eventually at 200 K, no change in M r could be observed ( Fig. 4b ). Therefore, a clear M–E hysteresis loop and non-volatile changes in M r seem to occur only when the transverse conical states is stabilized at zero H -bias. If the temperature to stabilize the transverse conical states at zero H -bias can be enhanced further, it is likely that the converse ME effects and its related mechanism, as observed here, could also be achieved even at higher temperatures. Figure 4: High-temperature modulation of magnetization under continuous and pulsed electric fields. ( a ) Δ M–E loops measured at 50, 100, 150 and 170 K. Hysteretic modulation was clearly observed up to 150 K (as high as 160 K). The central magnetization values at each temperature were found to be ~\n0.45, 0.48, 0.10, and 0.02 μ B per f.u., respectively, and this value was subtracted in each plot to more clearly display the magnetisation behaviour. ( b ) The non-volatile change in remanent M after the application of a short, triangular electric pulse with either a positive (red arrows) or negative (blue arrows) peak value of 4.2 MV m −1 , demonstrating that the M jumps occurred up to at least 150 K. The zero value at 200 K corresponds to the central magnetization value of 0.03 μ B per f.u. Full size image The M–H loops and 57 Fe NMR studies under electric-field bias To demonstrate the changing of M by E under finite H , we also measured the M–H loops under an E -bias, as shown in Fig. 2b . Overall, the magnetization curve varied under the application of a non-zero E bias for any given magnetic field, but the relative change was close to maximum at zero magnetic field. The coercive field under finite E was slightly reduced by ~\n10%, and the M–H curves slightly expanded sideways. Most notably, the M–H curves in Fig. 2b were found to be shifted by ~\n by an E of ±1.2 MV m −1 . These phenomena are very analogous to the usual exchange-bias effect, in which the shift of the central magnetic field occurs as if an internal H -bias were applied. In this case, E serves the same role as an internally applied magnetic field in the exchange-bias phenomena, such that a positive (negative) E results in a negative (positive) shift in the hysteresis loop, as if a positive (negative) H -bias had already been applied. This result implies that the role of the E -bias is equivalent to that of an H -bias itself. Therefore, it is expected that the effects of either an electric field or a magnetic field (although they are perpendicular) in this hexaferrite should be equivalent, and both should affect the clamped ferroelectric/ferrimagnetic domains. To further understand the microscopic origin of such changes in the M–H loop induced by E and the large converse effects observed in Figs 3 and 4 , we systematically studied the enhancement of the 57 Fe NMR signal intensity. When nuclear spins are excited by an oscillating magnetic field, they typically precess along the local magnetic field. In magnetic materials, the electron spins coupled with the nuclear spins via the hyperfine interaction in a magnetic domain also precess at the same frequency. This phenomenon generates an oscillating magnetic field that is much stronger than that generated by the nuclear spins only, resulting in an enhanced NMR signal [29] . The signal may also be enhanced in the domain wall, but such an enhancement occurs via a slightly different mechanism. Precessing nuclear spins in a domain wall cause the domain wall to be displaced back and forth at the same frequency. Then, the electron spins in the domain wall begin to oscillate, resulting in signal enhancement. Typically, the enhancement effect in the domain wall is larger than that in the domain. The inset of Fig. 5a presents the 57 Fe NMR spectra of Ba 0.5 Sr 1.5 Zn 2 (Fe 0.92 Al 0.08 ) 12 O 22 with and without E -bias at μ 0 H =0 mT. The directions of the fields are the same as in Fig. 2a , with an additional radio frequency (rf) magnetic field H rf along the ab plane. The NMR intensity was observed to change under external electric and magnetic fields, whereas the shape and position of the spectrum were not altered. In Fig. 5a,b , the signal intensities versus H rf are plotted for various H with and without E -bias for H rf || H and H rf ⊥ H , respectively. The overall intensity of the spectrum decreased with increasing H in both cases, which is consistent with general expectations because the presence of an external magnetic field prevents the magnetic moments of electrons from vibrating freely. However, we found that the enhancement effect was sensitive to the direction of H rf , as illustrated in Fig. 5c . The signal intensity decreased rapidly with H and disappeared above 50 mT for H rf || H , whereas it was much less sensitive for H rf ⊥ H . Because Ba 0.5 Sr 1.5 Zn 2 (Fe 0.92 Al 0.08 ) 12 O 22 is nearly in a single magnetic domain state at μ 0 H =50 mT, as can be inferred from Fig. 2b , this result suggests that the NMR signal obtained for H rf || H originated primarily from domain walls and that the signal obtained for H rf ⊥ H originated primarily from domains. 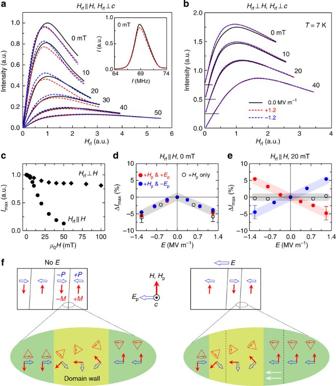Figure 5:The effects of magnetic and electric fields on the57Fe NMR signal and magnetic domain structure of Ba0.5Sr1.5Zn2(Fe0.92Al0.08)12O22. The NMR intensity versusHrfunder +Hp& +Epcondition for (a)Hrf||Hand (b)Hrf⊥H. The inset ofapresents the zero-field57Fe NMR spectrum. Inb, the data for μ0H=0 to 20 mT are shifted with respect to one another for clarity. The red dashed curves represent the data acquired under anE=+1.2 MV m−1, and the blue dashed curves correspond toE=−1.2 MV m−1. (c)Hdependence of the maximal signal intensity (Imax) in the absence ofE. (d,e)Edependence of the relative change in the maximal signal intensity (ΔImax) forHrf||Hat 0 and 20 mT. The red and blue solid circles represent data acquired after +Epand −Eppoling, respectively. The black open circles represent data acquired without ME annealing. All data were obtained at 7 K. (f) Schematic diagrams of changes in domain configuration withEandHunder the +Hp& −Epcondition. The directions of the ME annealing fields and thec-axis are the same as inFig. 2a. The two multiferroic domains hold for an orthogonal M and P relationship, and their domain walls move under the application of an externalE(white solid arrows), thus leading to an increase in the volume of one of multiferroic domains. Figure 5: The effects of magnetic and electric fields on the 57 Fe NMR signal and magnetic domain structure of Ba 0.5 Sr 1.5 Zn 2 (Fe 0.92 Al 0.08 ) 12 O 22 . The NMR intensity versus H rf under + H p & + E p condition for ( a ) H rf || H and ( b ) H rf ⊥ H . The inset of a presents the zero-field 57 Fe NMR spectrum. In b , the data for μ 0 H =0 to 20 mT are shifted with respect to one another for clarity. The red dashed curves represent the data acquired under an E =+1.2 MV m −1 , and the blue dashed curves correspond to E =−1.2 MV m −1 . ( c ) H dependence of the maximal signal intensity ( I max ) in the absence of E . ( d , e ) E dependence of the relative change in the maximal signal intensity (Δ I max ) for H rf || H at 0 and 20 mT. The red and blue solid circles represent data acquired after + E p and − E p poling, respectively. The black open circles represent data acquired without ME annealing. All data were obtained at 7 K. ( f ) Schematic diagrams of changes in domain configuration with E and H under the + H p & − E p condition. The directions of the ME annealing fields and the c -axis are the same as in Fig. 2a . The two multiferroic domains hold for an orthogonal M and P relationship, and their domain walls move under the application of an external E (white solid arrows), thus leading to an increase in the volume of one of multiferroic domains. Full size image The enhancement effect due to the rotation of the domain magnetization becomes maximal when H rf and the direction of magnetization in the domains are perpendicular to each other. On the other hand, the enhancement due to domain-wall movement is maximal when H rf and the direction of magnetization in the domains are parallel to each other because in this case, the domain walls can move more easily [30] . Therefore, the fact that the NMR signal primarily originates from domains for H rf ⊥ H and from domain walls for H rf || H means that the direction of magnetization in the domains is mostly parallel or antiparallel to H , and that the domain walls are parallel to H , as depicted in Fig. 5f . It is not surprising because of very small magnetic anisotropy in the plane for the transverse conical state (see Supplementary Fig. 2 ), although the hexagonal crystal symmetry predicts, in principle, three easy axes in the ab plane [31] . The most striking finding presented in Fig. 5a,b is that the signal intensity changed with E , either increasing or decreasing depending on the presence of H and the polarity of E . Fig. 5d,e illustrates the E dependence of the relative change in the maximal signal intensity (Δ I max ). At μ 0 H =0 mT ( Fig. 5d ), Δ I max decreased linearly with increasing E , irrespective of the direction of E p . Because the signal intensity is proportional to the domain-wall volume for H rf || H , a decrease in Δ I max indicates a domain-wall reduction induced by E ( Fig. 5f ). The non-poled sample (black open circles) exhibited nearly identical behaviour at μ 0 H =0 mT. At μ 0 H =20 mT ( Fig. 5e ), the application of an E in the opposite direction to E p partially recovered the intensity reduction caused by H , whereas the application of an E in the same direction further reduced the intensity. This behaviour can also be understood as a change in the domain-wall volume: An E in the same direction as the electric poling causes the domains whose orientations are parallel to H to expand, and consequently, the domain-wall volume is reduced. An E in the opposite to the direction of the electric poling produces the opposite effects. For the non-poled sample, Δ I max remained nearly constant, regardless of the electric-field direction. This finding suggests that half of the ferrimagnetic domains were coupled to the ferroelectric domains in the positive direction and the other half were coupled to the ferroelectric domains in the negative direction. This result is consistent with the observation that there are two different chiralities in the conical spin ordering of Ba 0.5 Sr 1.5 Zn 2 (Fe 0.92 Al 0.08 ) 12 O 22 , generating two opposite directions of electric polarization. All these results demonstrate, on the microscopic level, that the electric field plays a role equivalent to that of the magnetic field in changing the clamped ferrimagnetic/ferroelectric-domain configuration through the alignment of P and, consequently, M , thus revealing the microscopic origin of the strong cross-coupling effect observed in this hexaferrite. It is evident in Fig. 5b that the intensity of the NMR signal originating from the domains behaved quite differently from that of the signal originating from the domain walls. The NMR signal intensity always increased with increasing E , regardless of the poling direction. One possible explanation for this behaviour of the intensity originating from the domains is a change in the anisotropy field. The shrinkage of the coercive fields under the application of an E -bias in the M–H curves presented in Fig. 2b implies a small reduction of the magnetic anisotropy field. In such a case, the NMR signal is expected to be enhanced because magnetic anisotropy tends to fix the domain magnetisation along a certain direction, hindering magnetization rotation. Regardless of the mechanism, however, the change in the domain magnetization seems to be almost negligible compared with the gigantic converse ME coupling observed in Ba 0.5 Sr 1.5 Zn 2 (Fe 0.92 Al 0.08 ) 12 O 22 because the change is independent of the polarity of the applied electric field. Therefore, our NMR study demonstrates that the gigantic converse ME effect observed in Ba 0.5 Sr 1.5 Zn 2 (Fe 0.92 Al 0.08 ) 12 O 22 was accompanied by domain-wall movement induced by the electric field, originating from the strong clamping of the ferroelectric and ferrimagnetic domains created in the transverse conical spin state. The results of the NMR measurements of the zero-field-cooled sample are also consistent with this clamping picture, as the NMR signal intensity in this case exhibited no change with E within the experimental errors. It is because the longitudinal conical spin ordering ( Fig. 1b ), which forms after zero-field cooling, does not exhibit any ferroelectricity [25] . Rapid switching speed of M induced by E The NMR results implying the movement of magnetic domain walls under an electric field seem to be unique to this insulating helimagnet. As in the case of domain-wall motion driven by spin-transfer torque [32] , the domain-wall movement and the resultant changes in domain configuration under E in this compound might also be sufficiently rapid for practical application. To test how rapidly the magnetic domains and/or domain walls respond to an electric field, we measured the resistance change of a giant magnetoresistance (GMR) sensor glued to the bottom surface of the crystal under a rapid triangular E sweep, as depicted in Fig. 6a . We found that the GMR signals versus E exhibited nearly the same shape as the M–E loops presented in Fig. 3b , even when the E sweep frequency was varied from 1 to 10 kHz ( Fig. 6b ). When the sign of E p was reversed, the GMR signal versus E loops were modified accordingly, exhibiting behaviour very similar to that of the M–E loops presented in Fig. 3b . When the GMR signal versus time is plotted alongside the triangular E sweep applied on a time scale of ~\n30 μs (~\n10 kHz), it is clear that the curve closely follows the shape of the rapid E sweep ( Fig. 6c ). Although the speed of E could not be further increased because of the limitations of the electronics, this result indicates that the switching time of M induced by E has an upper limit of ~\n30 μs and may be much smaller than 30 μs. Our observation directly demonstrates that the speed of the domain-wall movement and the change in the domain configuration induced by E may be sufficiently rapid to be useful in practical applications. The present results also suggest that the microscopic coupling between electric field and spin configuration may allow the more rapid, electrical control of M in the frequency regime of giga or terahertz where the electromagnons of this helimagnet are located [33] . 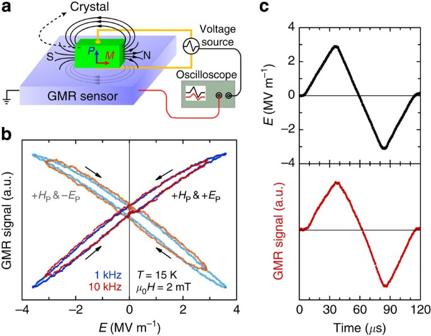Figure 6: Measurement of rapid magnetization change using a GMR sensor. (a) A schematic diagram of a Ba0.5Sr1.5Zn2(Fe0.92Al0.08)12O22single crystal bonded to the top of a GMR sensor. Electric pulses were applied sequentially while an oscilloscope was used to monitor the time dependence of the electric pulses and the changes in the voltage measured by the GMR sensor. (b)Edependence of the GMR signals at 15 K. The maximum modulation of the GMR signals under the electric-field sweep corresponds to an equivalent change in the magnetic field of ~\n2.5 mT. Note that the hysteresis in the plot of the GMR signal versus the electric field primarily originates from changes in the remanentM. (c) The full increase or decrease of the GMR signal occurs within ~\n30 μs, limited by the rise or fall time of the electric pulses, thereby indicating that the magnetization jumps can occur at least within 30 μs and possibly much more rapidly. Figure 6: Measurement of rapid magnetization change using a GMR sensor. ( a ) A schematic diagram of a Ba 0.5 Sr 1.5 Zn 2 (Fe 0.92 Al 0.08 ) 12 O 22 single crystal bonded to the top of a GMR sensor. Electric pulses were applied sequentially while an oscilloscope was used to monitor the time dependence of the electric pulses and the changes in the voltage measured by the GMR sensor. ( b ) E dependence of the GMR signals at 15 K. The maximum modulation of the GMR signals under the electric-field sweep corresponds to an equivalent change in the magnetic field of ~\n2.5 mT. Note that the hysteresis in the plot of the GMR signal versus the electric field primarily originates from changes in the remanent M . ( c ) The full increase or decrease of the GMR signal occurs within ~\n30 μs, limited by the rise or fall time of the electric pulses, thereby indicating that the magnetization jumps can occur at least within 30 μs and possibly much more rapidly. Full size image It is worth discussing the major properties of Ba 0.5 Sr 1.5 Zn 2 (Fe 0.92 Al 0.08 ) 12 O 22 that create favourable conditions for such a large converse ME effect. One of the key characteristics is likely to be the soft ferrimagnetism with very weak in-plane anisotropy that exists in the transverse conical state of this hexaferrite ( Supplementary Fig. 2 ). Unlike the conical spin state with an easy axis in CoCr 2 O 4 (ref. 26 ), our Ba 0.5 Sr 1.5 Zn 2 (Fe 0.92 Al 0.08 ) 12 O 22 has an easy ab plane after the field-cooling process, and the sixfold-hexagonal anisotropic energy seems to be almost negligible in the easy plane. The smaller the magnetic anisotropy is, the smaller is the energy that is required for the application of E to induce the simultaneous rotation of the P and M vectors inside the multiferroic domains or domain walls. Moreover, as implied in the ferroelectric phase diagram ( Supplementary Fig. 1 ), the transverse conical state at zero magnetic field in this annealed Ba 0.5 Sr 1.5 Zn 2 (Fe 0.92 Al 0.08 ) 12 O 22 seems to be stable up to ~\n150 K, below which temperature the converse ME effect becomes significant. Therefore, soft ferrimagnetism with minimal magnetic anisotropy and the related transverse conical spin state seems to be the most important factors leading to the observation of such large reversal and strong modulation of magnetization by an electric field. Furthermore, because other Y-type hexaferrites that exhibit a transverse conical state at higher temperatures exist, the mechanism and phenomena observed here are likely to be applicable even at room temperature [23] and thus may pave the way towards eventually utilizing gigantic converse ME effects in real devices at room temperature. Single-crystal growth and oxygen annealing Y-type Ba 0.5 Sr 1.5 Zn 2 (Fe 0.92 Al 0.08 ) 12 O 22 single crystals were grown from a Na 2 O-Fe 2 O 3 flux in air [34] . The chemicals were mixed with a molar ratio of BaCO 3 : SrCO 3 : ZnO: Fe 2 O 3 : Al 2 O 3 : Na 2 O=2.95: 16.74: 19.69: 49.32: 4.29: 7.01 and melted at 1420 °C in a Pt crucible, followed by several thermal cycles. The hexagonally-shaped single crystals of Ba 0.5 Sr 1.5 Zn 2 (Fe 0.92 Al 0.08 ) 12 O 22 were all grown in the same batch. The c- axis parameters of the crystals were determined using X-ray diffraction. To increase the resistivity of the specimens, an optimized heat-treatment process was applied, in which the temperature was maintained at 900 °C under flowing oxygen for 8 days, followed by cooling at a rate of 50 °C h −1 (ref. 35 ). ME annealing procedures The temperature and the magnetic field were controlled using a Physical Property Measurement System (PPMS; Quantum Design, USA). In all measurements, H was applied along the [100] direction, and E was applied along the [120] direction. For the electrical measurements, the samples were cut into a rectangular parallelepiped shape with the largest surface (~\n1 mm 2 ) normal to the [120] direction. Before the converse ME measurements, each specimen was subjected to an ME annealing procedure starting at 120 K. For the ME annealing condition of + H p & + E p , the sample was electrically poled at E =220 kV m −1 upon changing the magnetic field from the paraelectric collinear state (μ 0 H =2 T) to the ferrimagnetic state (μ 0 H =1.2 T) at 120 K. Then, with the same electric field and the magnetic field, the sample was initially cooled to the lowest investigated temperature (15 K). The E was then turned off at μ 0 H =1.2 T, the electrodes were shorted, and the magnetic field was ramped down to zero prior to the converse ME experiments. For the converse ME experiments at higher temperatures, we sequentially increased the temperature after performing the lower-temperature experiments at zero magnetic field. ME current measurements The ME current was measured and integrated to determine the change in the electric polarization with the magnetic field. For the ME current measurement at 15 K, a nearly identical ME annealing procedure was applied, except that the magnetic field was maintained at 1.2 T during the final stage. The ME current was then measured by sweeping H either to the outside or to the inside of the ferroelectric region by passing through the zero-field region, that is, either down to − 2 T or up to +2 T or first down to − 1.2 T and then up to +2 T. We also performed the equivalent converse ME and ME current experiments under the ME annealing condition of + H p , − E p in a similar manner. Magnetization under an electric field Magnetization curves were measured using a vibrating sample magnetometer (VSM) in a PPMS (Quantum Design). The sample was cooled from room temperature to 15 K at μ 0 H =2 T for the magnetization measurements after field cooling. For the magnetization measurements under an electric-field bias, we cooled the sample after applying the ME annealing procedure starting from 120 K as described above, and the target electric field was applied at 15 K and 1.2 T before ramping down the magnetic field. For the low- H measurements (|μ 0 H |≤2 mT) in particular, we carefully calibrated the H of the superconducting magnet in the PPMS using a standard paramagnetic Pd sample (Quantum Design Application Note 1070-207). For the magnetization measurements under E , we modified the conventional VSM sample holder to permit the application of high E . P–E loop measurements The P–E loop of the sample was measured using the Positive-Up-Negative-Down (PUND) method in our homemade setup to extract only the hysteretic parts of the change in the electric polarization [36] . Triangular electric pulses with a duration of 0.5 ms were applied, using a constant peak amplitude for each pulse. Ferroelectric phase diagram of the annealed crystal For Y-type multiferroic hexaferrites, oxygen annealing can slightly change the magnetic and ferroelectric phase boundaries [35] . Therefore, we determined the ferroelectric phase diagram of the studied crystals, in which the magnetization behaviour versus temperature indicated long-range antiferromagnetic ordering at the Néel temperature T N ~\n260 K. It is known that the ferroelectric phase diagram can be determined by measuring the dielectric anomaly (peak) as a function of the magnetic field under isothermal conditions [16] . By mapping out the peak field positions in the dielectric constant versus the magnetic field at selected temperatures, we plotted the ferroelectric phase diagram of the annealed crystals, as presented in Supplementary Fig. 1 . From this study, we found that the dielectric-constant peaks not only originate from switching at the paraelectric-to-ferroelectric phase boundary, but also appear at zero magnetic field upon the occurrence of field-induced ferroelectric-domain switching. In the transverse conical state that formed at zero H -bias after ME annealing, we observed a characteristic peak at zero magnetic field attributable to ferroelectric-domain switching up to ~\n150 K, in addition to the high-field peaks located above 1 T corresponding to the crossing of the paraelectric phase boundary. At ~\n150 K, the low-field peak slightly increased in magnetic field towards the 10–20 mT scale, and then, at higher temperatures, the peak structure broadened, indicating that the transverse conical state was only stable below 150 K at zero field. From a neutron-diffraction study [25] , we found that above 150 K, the alternating longitudinal conical state is stable up to around ~\n230 K at zero magnetic field. Between T N and 230 K, there seems to be a mixed phase that is a combination of a modified helix and alternating longitudinal conical states. Therefore, above ~\n150 K, there is no ferroelectric phase at zero magnetic field, and only a field-induced crossover from a paraelectric phase (longitudinal conical or modified helix phase) to a ferroelectric (transverse conical) phase seems to be gradually appearing. Magnetic anisotropy in Ba 0.5 Sr 1.5 Zn 2 (Fe 0.92 Al 0.08 ) 12 O 22 The transverse conical spin configuration in the Ba 0.5 Sr 1.5 Zn 2 (Fe 0.92 Al 0.08 ) 12 O 22 crystal has magnetic anisotropy of the easy-plane type in which magnetic anisotropy is very small. This feature can be demonstrated by handling the cone axis with a small rotating magnetic field of several tens of mT [17] . We demonstrated the angular dependence of P under rotating H of 20 mT, 0.2 T and 1 T applied in the ab plane, as illustrated in Supplementary Fig. 2 . All P -values followed nearly sinusoidal curves, strongly suggesting that the transverse cone axis follows the direction of H, while the spin helicity remains intact. The highly tunable P under the rotating H as small as 20 mT highlights the small magnetic anisotropy in the ab plane. NMR measurements The 57 Fe NMR spectra were obtained using our homemade spectroscopy setup and a standard spin-echo (π/2 − π) sequence. For H and E dependences of I max , the frequency of H 1 was 69 MHz, which was the central frequency of the main peak [37] . The ME annealing procedure for + H p & + E p was done as follows: the sample was cooled to 130 K in the absence of both H and E . At 130 K, the sample was electrically poled at E =250 kV m −1 while changing μ 0 H from 0 T to 0.4 T. Then, the sample was cooled to 7 K while both E and H turned on. GMR sensor measurements The GMR chip sensor (NVE Sensors, AA004-02) was calibrated at 15 K before we applied the electric field to the sample. To ensure operation in the linear region of the GMR sensor, a bias H of 2 mT was applied. Meanwhile, a constant excitation voltage of 0.4 V was applied to the GMR sensor during the measurements. The configuration of the sample was chosen such that the change in the direction of M was parallel to the H -sensitive direction of the GMR sensor. How to cite this article: Chai, Y. S. et al. Electrical control of large magnetization reversal in a helimagnet. Nat. Commun. 5:4208 doi: 10.1038/ncomms5208 (2014).